Depinning probability of a magnetic domain wall in nanowires by spin-polarized currents Current-induced magnetic domain wall motion is attractive for manipulating magnetization direction in spintronics devices, which open a new era of electronics. Up to now, in spite of a crucial significance to applications, investigation on a current-induced domain wall depinning probability, especially in sub-nano to a-few-nanosecond range has been lacking. Here we report on the probability of the depinning in perpendicularly magnetized Co/Ni nanowires in this timescale. A high depinning probability was obtained even for 2-ns pulses with a current density of less than 10 12 A m −2 . A one-dimensional Landau-Lifshitz-Gilbert calculation taking into account thermal fluctuations reproduces well the experimental results. We also calculate the depinning probability as functions of various parameters and found that parameters other than the coercive field do not affect the transition width of the probability. These findings will allow one to design high-speed and reliable magnetic devices based on the domain wall motion. Spin-transfer torque (STT) is of great technological interest as a tool to manipulate the magnetization direction of nanoscopic magnets [1] , [2] due to a potential to realize ultralow-power and high-performance integrated circuits [3] , [4] , [5] and storages [6] . There are mainly two ways to utilize the STT: one is current-induced magnetization switching (CIMS) in magnetic nanopillars [2] , [7] , [8] , [9] , [10] , [11] , [12] , and the other is current-induced domain wall motion (CIDWM) in magnetic nanowires [1] , [13] , [14] , [15] , [16] , [17] , [18] , [19] , [20] , [21] , [22] , [23] , [24] , [25] , [26] , [27] . In particular, the latter is promising for applications in which a domain wall (DW) moves numerous times within several nanoseconds’ duration [4] , or in which numerous DWs are shifted simultaneously [6] . As the key ingredient of these devices is current-induced displacement of DWs from one artificially prepared pinning site to another, it is very important to characterize the depinning properties, especially its probability and the relationship between the critical current and pulse duration in the nanosecond range. Whereas a theoretical model to address such issues for CIMS has been established [11] , [12] and confirmed in several experiments [7] , [9] , [10] , there has only been a few theoretical studies on CIDWM [16] , [17] . Here we show the DW depinning probability for various current pulse amplitudes and durations using an artificially prepared pinning site in magnetic nanowires. We observed DW depinning with a low error rate driven by nanosecond-long current pulses, suggesting suitability for the device application described above. Also, we elucidated a characteristic mechanism of the DW depinning, which is contrasting with the CIMS. Furthermore, we found that a theoretical model in which thermal fluctuations are taken into account showed good agreement with the experimental results. By using this model, we discuss the transition width of the depinning probability with various parameters. Sample structure and magnetic properties For DW depinning experiments, a perpendicularly magnetized Co/Ni multilayer [18] deposited onto a Si substrate was used. This is a promising material for application to DW-motion devices because of several features in terms of stable operation and retention characteristics [21] , [22] , [23] , owing to its nature that the DW can be driven by an adiabatic STT [22] . By measuring the magnetization curves of the blanket film along the in-plane and out-of-plane directions, the saturation magnetization M s , perpendicular anisotropy constant and coercive field were obtained to be 0.96 T, 6.1 × 10 5 J m −3 , and 16.5 mT, respectively, which are consistent with the values reported in previous works [21] , [22] , [23] , [24] . The deposited film was patterned into a cross-shaped nanowire with a 160-nm width, on which four Cr/Au electrodes (A–B, C, D, and E) were attached ( Fig. 1 ). The magnetization direction around the Hall cross of the nanowire was detected by measuring the Hall resistance through the extraordinary Hall effect. To prepare a DW in the nanowire, after saturating the magnetization with a large out-of-plane magnetic field, a current pulse was applied to the Cr/Au electrode (from A to B) under an out-of-plane assist field H a , where the current pulse generates a local Oersted field, which forms a reversal domain. All measurements were performed at room temperature. (See Fig. 1a for the experimental setup and Methods for detailed information about the sample preparation and measurement.) 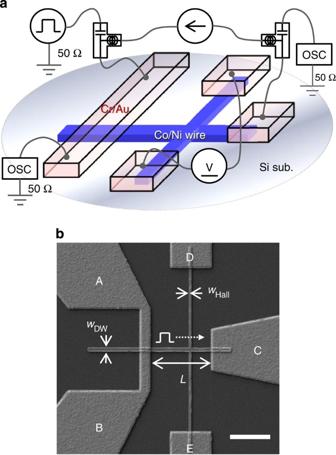Figure 1: Device structure and measurement circuit. (a) Schematic illustration of device structure with the measurement circuit used for DW depinning measurement. (b) Top view of a fabricated device taken by scanning electron microscope. Scale bar is 2 μm. Width of the DW-motion region,wDW, that of the Hall probe,wHall, and length between the interconnection A–B and electrode C,L, were designed to be 160 nm, 80 nm, and 3 μm, respectively. Figure 1: Device structure and measurement circuit. ( a ) Schematic illustration of device structure with the measurement circuit used for DW depinning measurement. ( b ) Top view of a fabricated device taken by scanning electron microscope. Scale bar is 2 μm. Width of the DW-motion region, w DW , that of the Hall probe, w Hall , and length between the interconnection A–B and electrode C, L , were designed to be 160 nm, 80 nm, and 3 μm, respectively. 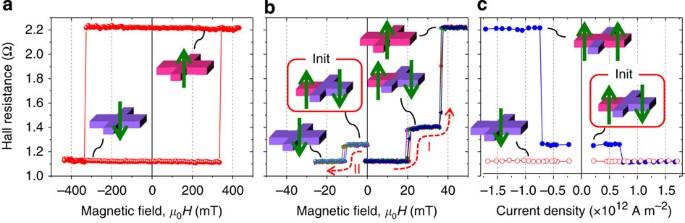Figure 2:R–HandR–jproperties. (a) MajorR–Hcurve. (b) MinorR–Hcurves obtained after DW injection. Resistance curves with positive field sweeping labelled I and negative field sweeping labelled II were obtained after an application of DW injection pulse at an assist fieldHaof 0 and +27 mT, respectively. Each measurement was repeated five times. (c) Variation of Hall resistance with current pulse application. Pulse current was applied with (closed blue symbols) and without (open red symbols) the DW preparation procedure. Schematic illustrations ina,bandcdepict the magnetic configuration for each resistance state. Full size image Figure 2a,b show resistance versus out-of-plane magnetic field ( R – H ) curves for the nanowire without and with DW, respectively. The insets illustrate the corresponding magnetization configurations. The major R – H curve in Fig. 2a shows a square hysteresis, indicating a perpendicular easy axis of the present Co/Ni nanowire. The coercive field, which corresponds to a nucleation field for magnetic domains, is about 350 mT. Figure 2b displays 10 independent R – H curves measured after preparing DW. The R – H curves obtained with no H a (labelled I) shows abrupt jumps at a sweeping field of about +20 and +35 mT. The former and latter fields correspond to a DW propagation field in the straight region and overpassing field to the right direction at the Hall cross, respectively [18] . On the basis of this result, the H a of +27 mT was used for initializing the DW at the left of the Hall cross, prior to all measurements of current-induced DW depinning described below. The negative field sweeping starting in this initial state (labelled II) shows a resistance drop at a field of about −12 mT. This field corresponds to the magnitude of the pinning potential formed at the left side of the Hall cross originating from the geometrical effect ( Supplementary Fig. S1 ) as well as pinning due to edge roughness and structural defects (see also Supplementary Note 1 in more detail); this field is different from the propagation field in the wire and coercive field of the blanket film. Figure 2: R – H and R – j properties. ( a ) Major R – H curve. ( b ) Minor R – H curves obtained after DW injection. Resistance curves with positive field sweeping labelled I and negative field sweeping labelled II were obtained after an application of DW injection pulse at an assist field H a of 0 and +27 mT, respectively. Each measurement was repeated five times. ( c ) Variation of Hall resistance with current pulse application. Pulse current was applied with (closed blue symbols) and without (open red symbols) the DW preparation procedure. Schematic illustrations in a , b and c depict the magnetic configuration for each resistance state. Full size image Current-induced DW depinning properties To examine the current-induced DW motion, the resistance versus current density ( R – j ) curve shown in Fig. 2c was measured by cycling through the following sequence: first, a DW was set at the initial site; second, a 10-ns-long current pulse with a variable amplitude and polarity was applied; third, the Hall resistance was measured. A positive (negative) current is defined as a current flowing from left (right) to right (left). The change in resistance without the DW preparation process was also measured as a reference (open symbols). In case that a DW was initialized, a positive (negative) current decreases (increases) the Hall resistance at an amplitude of more than ±7 × 10 11 A m −2 , whereas the resistance remains in the lowest state in case of no DW preparation procedure. This indicates that the DW trapped at the Hall cross was displaced by the applied current pulse in the direction of electron flow, which is consistent with the DW motion induced by STT. We evaluated the temperature increase due to Joule heating and found that it was as low as 20 °C at the current density of 1 × 10 12 A m −2 even in the dc case, suggesting that it is negligibly small in the present experiment using nanosecond pulses (see Supplementary Fig. S2 and Supplementary Note 2 ). Note also that the critical current density to move the DW to the right side becomes larger than that needed to move it to the left side as the pulse duration decreases to a few nanoseconds. This is due to a difference in pinning potential for the two DW motions, which will be discussed later. Hereafter, we will focus on DW depinning induced by a positive current injection, that is, depinning to the left direction from the Hall cross. 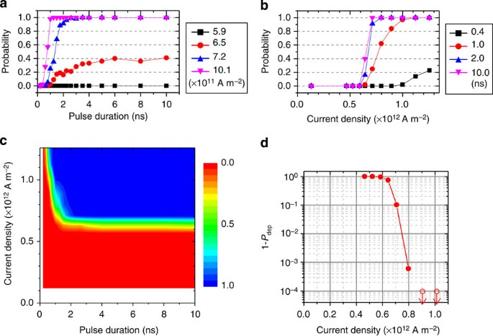Figure 3: Experimental results of DW depinning probability. (a)Pdepas a function of pulse duration for four current densities. (b)Pdepas a function of current density for four pulse durations. (c) Contour ofPdepwith current density and duration. (d) 1-Pdep, that is, depinning error rate, as a function of current density. The pulse duration was 2 ns. Experiment on DW depinning probability Figure 3 shows the DW depinning probability P dep for various current densities and pulse durations, where the rise and fall time of the pulse was less than 0.1 ns. To obtain P dep , the measurement was repeated 100 times for each condition. When the applied current density exceeds a certain threshold by about 10%, DW depinning becomes highly deterministic, that is, 100 successes for 100 trials, for pulse durations of more than about 2 ns, whereas no depinning was observed when the current density is less than the threshold by about 10% ( Fig. 3a ). Also, the transition of P dep from 0 to 1 with increasing current becomes steep when the pulse duration is longer than 2 ns ( Fig. 3b ). Interestingly, the critical current density with respect to the pulse duration is almost flat at durations longer than about 2 ns, whereas it significantly increases for durations less than 2 ns ( Fig. 3c ). We will discuss the relationship between the critical current density and pulse duration later. Figure 3d shows 1- P dep , that is, the depinning error rate, obtained by 10 4 repetitions with the same measurement sequence for 2-ns-long current pulses with various amplitudes. A slight increase in current density above a certain threshold results in a steep decrease in the error rate. It is also notable that no error was observed in 10 4 trials when the current density exceeds 8.5 × 10 11 A m −2 . Figure 3: Experimental results of DW depinning probability. ( a ) P dep as a function of pulse duration for four current densities. ( b ) P dep as a function of current density for four pulse durations. ( c ) Contour of P dep with current density and duration. ( d ) 1- P dep , that is, depinning error rate, as a function of current density. The pulse duration was 2 ns. Full size image Calculation of DW depinning probability Let us consider the model describing the DW depinning probability shown in Fig. 3 . In order to reproduce the stochastic nature of DW depinning, we took into consideration thermal fluctuations, which have also been considered for describing CIMS at a finite temperature [11] , [12] . We used the one-dimensional Landau-Lifshitz-Gilbert equation, in which the state of the DW is expressed by two collective coordinates ( q , ϕ ) representing the position and phase of the DW, and calculated the dynamics of a DW depinned from a parabolic pinning potential [25] , ( Fig. 4a ), (see Supplementary Note 3 ). The effect of thermal fluctuations was included as a distribution of initial ( q , ϕ ) values (see Supplementary Note 4 ) and a random magnetic field that satisfies the fluctuation-dissipation theorem [28] , (see Supplementary Note 5 ). We set each parameter so as to match the present Co/Ni system (see Methods for details). 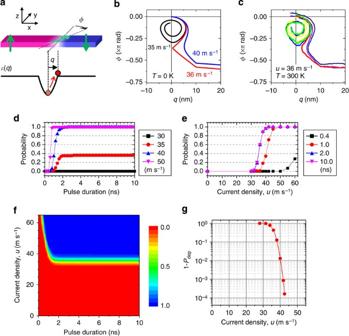Figure 4: Calculation result of DW depinning probability. (a) Definition of parameter (q,ϕ) used in one-dimensional LLG calculation.qis the position in relation to the pinning centre andϕis angle of the DW magnetization, where magnetization points in the transverse direction relative to the wire, that is, the Bloch wall state, is defined asϕ=0. (b) Trajectory of (q,ϕ) during current-induced DW depinning without thermal fluctuation. Trajectories with three current density values are shown. (c) Trajectory of (q,ϕ) with the thermal fluctuation. Six trajectories with the same current density are shown. (d)Pdepas a function of pulse duration for four current densities. (e)Pdepas a function of current density for four pulse durations. (f) Contour ofPdepwith current density and duration. (g) 1-Pdep, that is, depinning error rate, as a function of current density. The pulse duration was 2 ns. To obtainPdep, the calculation was iterated 100 times for (d–f) and 25,000 times for (g). Figure 4: Calculation result of DW depinning probability. ( a ) Definition of parameter ( q , ϕ ) used in one-dimensional LLG calculation. q is the position in relation to the pinning centre and ϕ is angle of the DW magnetization, where magnetization points in the transverse direction relative to the wire, that is, the Bloch wall state, is defined as ϕ =0. ( b ) Trajectory of ( q , ϕ ) during current-induced DW depinning without thermal fluctuation. Trajectories with three current density values are shown. ( c ) Trajectory of ( q , ϕ ) with the thermal fluctuation. Six trajectories with the same current density are shown. ( d ) P dep as a function of pulse duration for four current densities. ( e ) P dep as a function of current density for four pulse durations. ( f ) Contour of P dep with current density and duration. ( g ) 1- P dep , that is, depinning error rate, as a function of current density. The pulse duration was 2 ns. To obtain P dep , the calculation was iterated 100 times for ( d – f ) and 25,000 times for ( g ). Full size image Figure 4b,c show the trajectories of ( q , ϕ ) after the current is turned on without and with thermal fluctuations, respectively. With the present set of parameters, the critical current density u c is 36 m s −1 at 0 K ( Fig. 4b ). Figure 4c shows six independent calculation results where the current density and temperature T were 36 m s −1 and 300 K. Three of those are depinned while the others are not; this shows the stochastic nature of DW depinning. Also, looking carefully at the trajectories, we can see that both the initial distribution of ( q , ϕ ) and disturbance during the time evolution of ( q , ϕ ) affect whether the DW can be depinned. For example, DWs starting with a positive ϕ generally tend to be depinned, but the trajectory shown by the green curve shows no depinning, although its initial state is similar to the red curve, which shows depinning. Figure 4d–g are the calculation results corresponding to Fig. 3a–d , respectively. It is clear that the calculation well reproduces the tendencies observed in our experiment; for example, the critical current density is almost constant when the pulse duration is above 2 ns, and the error rate steeply decreases when the current density is slightly larger than a certain threshold value. First, we should note the good agreement between the experiment and the calculation. This allows us to evaluate the DW depinning properties at a finite temperature, as described below. Based on the above model, we calculated the DW depinning probability with various parameters ( Supplementary Fig. S3 ). We found that size of the pinning potential q 0 and intrinsic pinning field H c0 influence only the horizontal scale of the P dep contour; for example, the pulse duration above which the critical current density is almost constant increases with q 0 . On the other hand, the hard-axis anisotropy field H k and DW width parameter Δ influence only the vertical scale, and the Gilbert damping constant α and non-adiabatic coefficient β have limited influence on the DW depinning properties. We also examined the transition width of P dep . 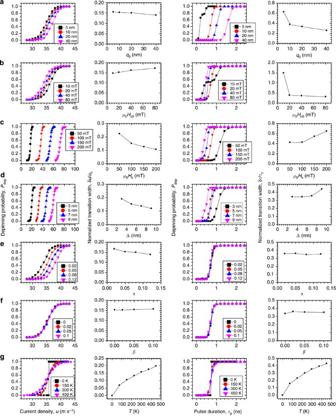Figure 5: Transition ofPdepfor various parameters. The first column shows,Pdepversus current densityu.; the second column, the transition width ofPdepwith respect to the current density δunormalized by the critical current densityuc, (δu/uc), as a function of each parameter; the third column,Pdepversus pulse durationτp; and the fourth column the transition width ofPdepwith respect to the pulse duration δτnormalized by the critical pulse durationτc, (δτ/τc), as a function of each parameter. For the first and second columns, the pulse duration was fixed to 5 ns. δu(δτ) was defined as the difference betweenu(τ) forPdep=10% and 90%.uc(τc) was defined as theu(τ) forPdep=50%. These parameters are presented as a function of (a) pinning potential sizeq0, (b) intrinsic critical fieldHc0, (c) hard-axis anisotropy of DWHk, (d) domain wall width parameter Δ, (e) Gilbert damping constant α, (f) non-adiabatic coefficientβand (g) temperatureT. Figure 5 shows P dep and its transition width with respect to the current density and pulse duration for various parameters calculated from 500 iterations. The transition width of P dep is strongly affected by T ( Fig. 5g ). In addition, when H c0 is so small that the length scale of the motion of the DW in the potential well reaches q 0 , the transition width with respect to the pulse duration significantly increases ( Fig. 5b ). The other parameters studied here do not prominently affect the transition width. Furthermore, the characteristics of the P dep contour remain virtually unchanged even though these parameters vary by a factor of 2. Such features can be attributed to the DW depinning process being driven by an adiabatic spin-transfer torque in the so-called intermediate regime, where the threshold of the depinning is determined by the hard-axis anisotropy [19] . We also note that, because the numerically calculated μ 0 H c0 , which gives the upper limit of the intermediate regime, is as large as 2 T, practically all realistic experimental conditions fall within this regime. Therefore, the present findings cover the entire experimentally accessible range and allow one to employ a wide variety of materials, because they do not affect the stable operation of the DW-motion devices. Figure 5: Transition of P dep for various parameters. The first column shows, P dep versus current density u . ; the second column, the transition width of P dep with respect to the current density δ u normalized by the critical current density u c , (δ u / u c ), as a function of each parameter; the third column, P dep versus pulse duration τ p ; and the fourth column the transition width of P dep with respect to the pulse duration δ τ normalized by the critical pulse duration τ c , (δ τ / τ c ), as a function of each parameter. For the first and second columns, the pulse duration was fixed to 5 ns. δ u (δ τ ) was defined as the difference between u ( τ ) for P dep =10% and 90%. u c ( τ c ) was defined as the u ( τ ) for P dep =50%. These parameters are presented as a function of ( a ) pinning potential size q 0 , ( b ) intrinsic critical field H c0 , ( c ) hard-axis anisotropy of DW H k , ( d ) domain wall width parameter Δ, ( e ) Gilbert damping constant α, ( f ) non-adiabatic coefficient β and ( g ) temperature T . Full size image Next, let us examine the relationship between the critical current density j c and pulse duration τ p , by comparing the experimental results with the calculation in more detail. 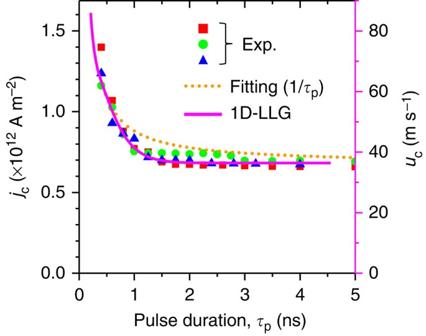Figure 6: Relation betweenjcandτp. Experimental results for the critical current densityjc, as a function of pulse duration for three different devices (red squares, green circles and blue triangles). Curve fitted to the experimental data with the inverse relation,jc−jc01/τp(dotted line) and one-dimensional LLG calculation (solid line). The right vertical axis (uc) is for the one-dimensional LLG calculation, whereas the left vertical axis (jc) is for the other data. Figure 6 shows the experimentally obtained j c as a function of τ p for three different devices with the same structure. Here, j c is defined as the current density that gives P dep =0.5. One can see that the dependence of j c on τ p is quite similar among the three devices. The fitting curve with the inverse relation, that is, j c — j c0 1/ τ p , which is true for CIMS in nanopillars [7] , [9] , [11] , is also shown in the figure (dotted line). This relation is based on magnetization reversal originating from the current-induced torque through conservation of spin angular momentum [7] . In addition, a result of a one-dimensional Landau-Lifshitz-Gilbert calculation is shown (solid line). It is apparent that the inverse relation poorly fits the experimental results, whereas the numerical calculation agrees well with them. The discrepancy from the inverse relation can be accounted for in terms of the characteristic mechanism of DW depinning by adiabatic STT. In the adiabatic regime, a DW can be depinned when Walker breakdown occurs. Here, not only STT but also the effective field originating from the pinning potential has a significant role in inducing Walker breakdown [19] , [20] . Consequently, the depinning time is not simply proportional to the inverse of the current (see Supplementary Fig. S4 and Supplementary Note 6 in more detail). This is why the critical current density does not increase as the pulse duration decreases down to about 2 ns, and a low error rate is possible even at a current density of less than 10 12 A m −2 . The fact that j c does not increase down to about 2 ns is favourable for DW-motion devices with an operation frequency of several hundred MHz. Similarly, the steep decrease in the error rate above the threshold is promising to achieve reliable devices operated at a high working rate. It should also be noted that these features are in stark contrast to the case of CIMS in nanopillars, where j c is inversely proportional to τ p and the logarithm of the switching error rate almost linearly decreases as the current density increases in a-few-nanosecond, that is, precessional, range. Figure 6: Relation between j c and τ p . Experimental results for the critical current density j c , as a function of pulse duration for three different devices (red squares, green circles and blue triangles). Curve fitted to the experimental data with the inverse relation, j c − j c0 1/ τ p (dotted line) and one-dimensional LLG calculation (solid line). The right vertical axis ( u c ) is for the one-dimensional LLG calculation, whereas the left vertical axis ( j c ) is for the other data. Full size image In summary, we investigated the DW depinning probability both experimentally and theoretically. The experimental results indicate that highly deterministic DW depinning is possible with a nanosecond-long current pulse, suggesting a potential for device applications with high-speed driving of DWs at low error rates. Moreover, the theoretical model we used describes well the experimental results and gives us useful information for developing current-induced DW-motion devices. Film deposition The Co/Ni multilayer was deposited on a highly resistive Si substrate with a natural oxidation layer at room temperature through dc magnetron sputtering. The stack structure was, from the substrate side, Ta(3.0)/Pt(2.0)/[Co(0.3)/Ni(0.6)] 4 /Co(0.3)/Pt(1.5)/Ta(3.0) (in nanometres). Device fabrication The Co/Ni multilayer was patterned into cross-shaped nanowires by using electron beam lithography and Ar ion beam milling. Cr(5)/Au(100) electrodes were formed onto the Co/Ni nanowire by using electron beam lithography and lift-off. Hall measurement The Hall resistance was evaluated by measuring the voltage between electrodes D and E upon application of a 50 μA dc current (4.2 × 10 10 A m −2 ) between electrodes A and C in Fig. 1b . R – H curves measurement after DW injection The two types of R – H curve shown in Fig. 2b were obtained through the following sequence: (1) apply a magnetic field of −500 mT to align all magnetizations in the downward direction; (2) inject a current pulse with an amplitude of about 150 mA and duration of 10 ns from electrodes A–B to nucleate an upward magnetic domain in the vicinity of the interconnection under an assist field H a ; (3) measure the Hall resistance by sweeping the magnetic field in the positive or negative direction. Numerical calculation The parameters used for the numerical calculation were set according to the present Co/Ni wire. The actual values are as follows: w =160 nm, t =3.9 nm, α=0.05 (ref. 29) [29] , β =0.02 [26] (ref. 26), Δ =5.4 nm, which was derived from a two-dimensional micromagnetic simulation, μ 0 H k =100 mT, which was also derived from a two-dimensional micromagnetic simulation, μ 0 H c0 =20 mT, which was determined from the experimental result shown in Fig. 2b with taking the effect of thermal fluctuation into account, and q 0 =10 nm (see Supplementary Fig. S1 and Supplementary Note 1 ). T was 300 K. The actual form of the random magnetic field H rand derived from the fluctuation-dissipation theorem is , where the time step of the application of the random magnetic field d τ was set to be 1 ps (see Supplementary Note 5 ). How to cite this article: Fukami, S. et al. Depinning probability of a magnetic domain wall in nanowires by spin-polarized currents. Nat. Commun. 4:2293 doi: 10.1038/ncomms3293 (2013).